An invisible acoustic sensor based on parity-time symmetry Sensing an incoming signal is typically associated with absorbing a portion of its energy, inherently perturbing the measurement and creating reflections and shadows. Here, in contrast, we demonstrate a non-invasive, shadow-free, invisible sensor for airborne sound waves at audible frequencies, which fully absorbs the impinging signal, without at the same time perturbing its own measurement or creating a shadow. This unique sensing device is based on the unusual scattering properties of a parity-time (PT) symmetric metamaterial device formed by a pair of electro-acoustic resonators loaded with suitably tailored non-Foster electrical circuits, constituting the acoustic equivalent of a coherent perfect absorber coupled to a coherent laser. Beyond the specific application to non-invasive sensing, our work broadly demonstrates the unique relevance of PT-symmetric metamaterials for acoustics, loss compensation and extraordinary wave manipulation. When we measure a physical quantity of interest, we intrinsically perturb its spatial distribution, creating reflections and a shadow associated with the energy extracted by our measurement. The larger the signal we pick up with our sensor, the more the wave scattering we typically generate. It has been recently suggested that this problem may be overcome using metamaterial cloaks, which may avoid the scattering of a sensor, while at the same time maintaining its ability to receive energy from the surroundings [1] , [2] , [3] . However, power conservation arguments require that any passive object is bound to generate a finite shadow proportional to the amount of absorbed energy, and low scattering can only be achieved at the price of reduced absorption [4] . This trade-off and limitation may be lifted by considering active systems. In a seemingly unrelated area of modern theoretical physics, significant attention has been devoted to non-Hermitian Hamiltonians H that commute with the parity-time (PT) operator, a property that can lead to real-energy eigenvalues [5] , [6] . Translated to optics, it has been theoretically argued that PT-symmetric systems, obtained with properly balanced distributions of absorbing and gain media, may produce lossless propagation [7] , [8] , [9] , [10] , [11] , remarkably opening paths to loss compensation [12] , [13] , [14] , [15] , [16] , [17] , [18] and, under special conditions, unidirectional invisibility in one-dimensional systems [17] , [18] , a phenomenon also known as anisotropic transmission resonance (ATR) [14] . Experimental investigations of these exotic scattering phenomena have been so far quite limited, conducted in the temporal domain [19] , [20] , [21] , or in the spatial domain for passive (that is, non-fully-PT-symmetric) [22] , [23] and active [11] , [24] , [25] spatial distributions of refractive index. Here we observe these properties for sound waves, and use PT symmetry to realize a non-invasive, shadow-free, fully invisible acoustic sensor, based on a PT-symmetric distribution of balanced gain and loss. Our experiment also constitutes direct experimental evidence of PT-symmetric unidirectional invisibility in acoustics, and highlights its remarkable implications for non-invasive sensing. The proposed concept is schematically represented in Fig. 1 : in order to extract energy from the incoming sound wave, we use a conventional acoustic sensor (left element in Fig. 1a ), in the form of a loudspeaker connected to an electric circuit with passive impedance , tailored to absorb a portion of the impinging signal. This sensor, operated by itself, would inherently produce a shadow associated with the power that it absorbs, as well as some reflections and scattering. In order to realize an invisible sensing device, without reflections or shadows, we place a second loudspeaker at distance d from the first one (right element in Fig. 1a ), loaded with an active electrical circuit tailored to realize the time-reversed image of the left loudspeaker. The original sensor, which is still capable of absorbing power, is now used as the lossy constituent of a PT-symmetric system with balanced loss and gain. By operating the PT system in the non-trivial ATR condition [14] , shown in the figure, we obtain a unique device that, while being capable of strongly sensing a signal via its passive component, is also totally invisible. More specifically, this PT metamaterial cell lets the acoustic energy flow totally undisturbed, without reflections or shadows, when excited from the left ( Fig. 1a ): while the first (sensing) loudspeaker absorbs the impinging energy, the second (active) loudspeaker restores the energy balance. Note that such power compensation process is obtained between two elements that are electrically disconnected, and that interact only through scattering. When excited from the active side, such a device is instead strongly reflective ( Fig. 1b ), consistent with the asymmetric response typically expected in PT-symmetric systems operated in the non-trivial ATR condition. 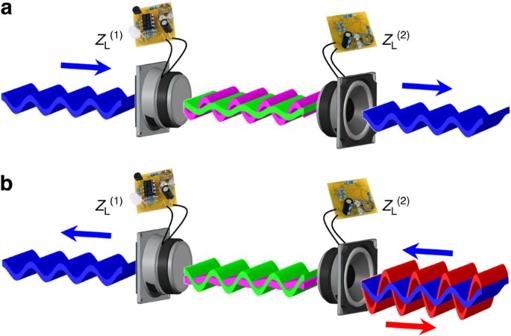Figure 1: A parity-time invisible acoustic sensor. A PT-symmetric acoustic system is realized by using a pair of electromechanical resonators (here loudspeakers) loaded with properly tailored electrical circuits. The left loudspeaker is operated as a sensor by loading it with an absorptive circuit, while the other forms an acoustic gain element. Their combination is a compact PT-symmetric unit cell that is transparent from the left (a), while it can at the same time extract the impinging signal. On the contrary, the system is highly reflective when excited from the right (b). Figure 1: A parity-time invisible acoustic sensor. A PT-symmetric acoustic system is realized by using a pair of electromechanical resonators (here loudspeakers) loaded with properly tailored electrical circuits. The left loudspeaker is operated as a sensor by loading it with an absorptive circuit, while the other forms an acoustic gain element. Their combination is a compact PT-symmetric unit cell that is transparent from the left ( a ), while it can at the same time extract the impinging signal. On the contrary, the system is highly reflective when excited from the right ( b ). Full size image Theory As a proof of concept, we consider a PT-symmetric invisible sensor enclosed in an acoustic waveguide consisting of a straight air-filled pipe with hard solid walls. The loudspeakers may be modeled as transverse mechanical resonators, which modify the local effective density of the acoustic medium with minimal effects on its effective bulk modulus [26] ( Supplementary Note 1 ). We tailor the circuit impedance loading the two loudspeakers to synthesize a one-dimensional acoustic metamaterial cell whose effective density distribution ρ ( z ) has a homogeneous real part equal to the background density ρ 0 , while its imaginary part follows the odd-symmetric distribution ( Fig. 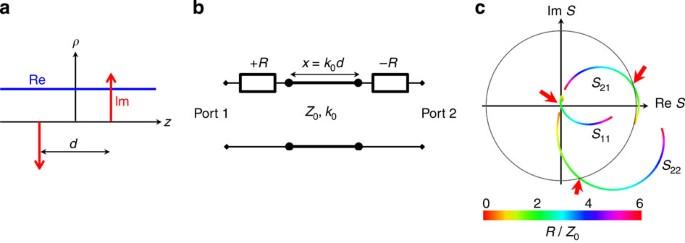Figure 2: Scattering properties. (a) Desired PT-symmetric density distribution. (b) Two-port transmission-line model of the acoustic system ofFig. 1, composed of two lumped elements with resistance +Rand −R, separated by a portion of transmission line of acoustic lengthxand characteristic impedanceZ0. (c) Scattering parameters as a function of the parameterr=R/Z0, forx=sin−1(1/4). A unidirectional invisible device is obtained forr=2 (red arrows). 2a ): Figure 2: Scattering properties. ( a ) Desired PT-symmetric density distribution. ( b ) Two-port transmission-line model of the acoustic system of Fig. 1 , composed of two lumped elements with resistance + R and − R , separated by a portion of transmission line of acoustic length x and characteristic impedance Z 0 . ( c ) Scattering parameters as a function of the parameter r = R / Z 0 , for x =sin −1 (1/4). A unidirectional invisible device is obtained for r =2 (red arrows). Full size image Since both P and T operators have the effect of switching the sign of the imaginary part of the density, it is easily seen that this spatial distribution is indeed PT-symmetric, as desired. Such a unit cell can be modelled using an equivalent two-port transmission-line model, as in Fig. 2b . The loudspeakers are represented as series lumped elements, surrounded by transmission-line segments of impedance , representing the waveguide portions, with κ 0 being the background bulk modulus and S 0 the waveguide cross-section. The acoustic separation length is x = k 0 d , where k 0 is the free-space wave number. In order to synthesize the effective density distribution (1), the loading circuits should be chosen such that the first loudspeaker is characterized by a passive acoustic resistance R = ρ L ω / S 0 ( Supplementary Note 1 ), while the second one supports acoustic gain with negative resistance − R . This requires the use of active circuitry, implemented here using non-Foster circuit elements, which have recently become of interest in antenna systems [27] and metamaterial technology [28] , [29] . Such active circuit elements are suitably designed here to guarantee full acoustic stability, avoiding unwanted oscillations. The scattering matrix of the metamaterial cell in Fig. 2b can be calculated using a transmission-matrix approach ( Supplementary Note 2 ): where r = R / Z 0 . It is straightforward to verify that S indeed possesses the special symmetry PT S ( ω *) PT = S −1 ( ω ), as expected for PT symmetric systems [14] . Equation (2) describes a reciprocal and linear system that possesses interesting scattering properties as a function of the values of r and x . Figure 2c , for instance, shows the effect of varying r = R / Z 0 on the evolution of the scattering parameters in the complex plane for x =sin −1 (1/4). The colours show the scattering evolution as the parameter r is varied, as indicated in the legend. A condition of special interest is given by r =2 (highlighted in Fig. 2c by red arrows), for which we obtain unidirectional transparency, or non-trivial ATR, with zero reflection at port 1 ( S 11 =0), unitary reflection at port 2 (| S 22 |=1, Supplementary Fig. 1 ) and unitary transmittance at both ports | S 12 |=| S 21 |=1. In Supplementary Note 3 , we study the spectral properties of the S matrix, showing that this condition does not arise at the spontaneous PT-symmetry breaking ( Supplementary Fig. 2 ), but corresponds to an exceptional point, for which the spectrum of the transformed matrix Sσ 1 , with σ 1 ={{0, 1}; {1, 0}} being the first Pauli matrix, escapes the unitary complex circle [14] . This unidirectional reflectionless response is actually independent of the distance x , as can be seen by evaluating the scattering matrix (2) for r =2: Such a system therefore realizes an acoustic sensor that is ideally invisible when excited from one side, with no reflections and unitary transmission independent of the electrical distance x between the two subunits, but that at the same time strongly reflects when excited from the other side, consistent with the sketch in Fig. 1 . The passive (left) portion of the device efficiently absorbs the impinging signal, while the active (right) portion provides the required energy to suppress any shadow. It is worth pointing out here that transmission is accompanied by a phase advance that is exactly opposite to the phase the wave would acquire over the distance x in the background medium. This implies that, as a by-product of our furtive sensor design, we also obtain an effective impedance-matched, negative-index metamaterial unit cell for arbitrary distance x . In addition to being used for furtive sensing, such a cell may be used in arrays to achieve negative refraction for sound in a metamaterial-free, loss-immune fashion, extending the findings in ref. 30 to acoustic waves. PT acoustic metamaterial cell and its operation Because of the appealing scattering features occurring at the exceptional point r =2, we tailored our two loudspeakers and their circuit loads to fulfill this condition at their resonance frequency f r =250 Hz. The geometry, materials and design procedures of the PT-symmetric metamaterial cell are detailed in the Methods section. The normalized acoustic impedance of the loaded loudspeaker at port 1 is shown in Fig. 3a as a function of frequency, and that of the second loudspeaker in Fig. 3b . At f r =250 Hz the acoustic impedance of the first loudspeaker is exactly twice the line impedance, with no imaginary part, and the one at port 2 is the opposite, satisfying the condition r =2 for unidirectional invisibility. The dispersion of the − R loudspeaker, which follows an inverted Lorentzian profile typical of gain media ( Fig. 3b ), is tailored by a non-Foster circuit to ensure stability, by carefully positioning the zeros and poles of its electrical load in the complex plane ( Supplementary Fig. 5 ). The separating distance x =sin −1 (1/4) has been chosen to ensure unitary reflection at port 2, consistent with equation (3). 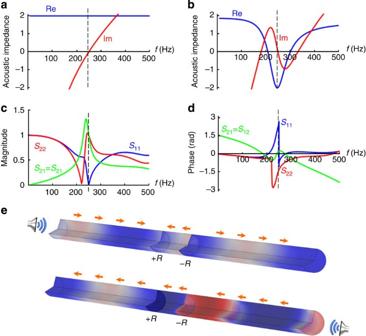Figure 3: Expected scattering properties of the PT-symmetric acoustic element. Frequency dispersion of the normalized acoustic impedance of the loudspeakers at ports 1 (a) and 2 (b), showing that the exceptional point conditionr=2 for unidirectional invisibility is achieved atf=250 Hz (dashed vertical line). (c,d) Scattering parameters (analytical) as a function of frequency, magnitude (c) and phase (d). Atf=250 Hz (dashed vertical line), the reciprocal device shows zero reflection and unitary power transmission from port 1. From port 2, however, reflection is unitary. (e) Acoustic pressure distribution atf=250 Hz for excitation from port 1 (top) and from port 2 (bottom), from full-wave FEM simulations. The arrows represent the direction of average power flow along the waveguide. Figure 3: Expected scattering properties of the PT-symmetric acoustic element. Frequency dispersion of the normalized acoustic impedance of the loudspeakers at ports 1 ( a ) and 2 ( b ), showing that the exceptional point condition r =2 for unidirectional invisibility is achieved at f =250 Hz (dashed vertical line). ( c , d ) Scattering parameters (analytical) as a function of frequency, magnitude ( c ) and phase ( d ). At f =250 Hz (dashed vertical line), the reciprocal device shows zero reflection and unitary power transmission from port 1. From port 2, however, reflection is unitary. ( e ) Acoustic pressure distribution at f =250 Hz for excitation from port 1 (top) and from port 2 (bottom), from full-wave FEM simulations. The arrows represent the direction of average power flow along the waveguide. Full size image The S -parameters of this PT acoustic device, based on our theory, are shown in Fig. 3c,d as a function of frequency. Figure 3c shows the magnitude of S 11 , S 22 and S 21 = S 12 , and Fig. 3d shows the associated phase. At f r =250 Hz (vertical dashed line), the system is indeed unidirectionally invisible, with S 11 =0, | S 22 |=| S 21 |=1, and it features the aforementioned anomalous phase advance at the transmission side. Note that the bandwidth of operation, which is relatively narrow here, may be in principle increased by engineering the dispersion of the electrical loads around the frequency of operation, adopting a more complex circuit design. Along this line, properly tailored non-Foster circuits have been recently envisioned for broadband metamaterial operation [31] . To validate this unusual scattering response and gain further physical insights into the operation of this device, we have performed full-wave simulations of the PT-symmetric acoustic cell in Fig. 1 using COMSOL Multiphysics, carefully modelling the acoustic inclusions by coupling acoustic and electrical circuit modules. The agreement between analytical ( Fig. 3c,d ) and full-wave simulation results ( Supplementary Fig. 6 ) is excellent. Figure 3e shows the acoustic pressure distribution in the device (snapshot in time) when excited at f =250 Hz by a wave incident from ports 1 (top) and 2 (bottom). From port 1, the incident wave is transmitted through the structure with the expected phase advance, no attenuation and zero reflection. From port 2, the wave is transmitted to port 1 with same amplitude and phase, consistent with reciprocity, but an additional strong reflection arises at this port, associated with a large standing wave ratio. We also plot the direction of average power flow in the system, represented by the orange arrows in the figure. Quite interestingly, the backward phase flow between the two loudspeakers, which is associated with the predicted phase advance, is sustained by a negative power flow, fed by the active inclusion, a unique feature of this PT negative-index metamaterial cell. At the sensing loudspeaker, the incident signal and the wave fed by the active inclusion add up in phase, and they are both completely absorbed by the passive loudspeaker, which forms the acoustic equivalent of a coherent perfect absorber [32] , or a time-reversed lasing system, capable of absorbing all the incident power, as well as the power travelling backward from the active loudspeaker, without reflections. The power absorbed by the loudspeaker is then exactly twice the incident power, in total contrast with passively cloaked sensors, which typically absorb a very small portion of the incident signal. The right loudspeaker, on the contrary, is the acoustic equivalent of a coherent laser, which emits a signal perfectly synchronized in phase and amplitude with the impinging signal. While the backward portion of the emitted signal feeds the passive loudspeaker, the forward portion is responsible for eliminating the shadow, making the PT metamaterial cell fully invisible. It is remarkable that the synchronization between the impinging signal and the active loudspeaker automatically takes place in free space through airborne sound waves: the loss and gain elements of the sensor are indeed totally independent electrically, and connected only via scattering. Such an exotic response can only be understood as a consequence of PT symmetry. Experimental validation A picture of the fabricated PT acoustic device is shown in Fig. 4a , showing the two loudspeakers separated by a 5.5-cm-long portion of a square acoustic waveguide. The non-Foster electrical circuits used to load the loudspeakers are implemented on a prototyping board with off-the-shelf electrical components, which can be manually tuned to ensure that the device is set to r =2 at the design frequency. Note that the specific orientation of the loudspeakers does not matter at such a subwavelength scale, and was chosen to be different from that in Fig. 1 for experimental convenience. In addition, we stress that, while the two electrical loads have been implemented on the same prototyping board for compactness, they are completely independent and electrically disconnected. The PT acoustic system is placed between two waveguides, as shown in Fig. 4b , and its scattering parameters are measured using the calibration procedure described in the Methods section. We excite the structure with a sinusoidal sweep, and measure the scattering parameters, which are shown in Fig. 5a (magnitude) and Fig. 5b (phase), in excellent agreement with the theoretical predictions of Fig. 3 . The fabricated device is indeed unidirectionally invisible at the design frequency (vertical dashed line), and we also measured the correct phase advance e jx for the transmitted signal, in agreement with the theory. 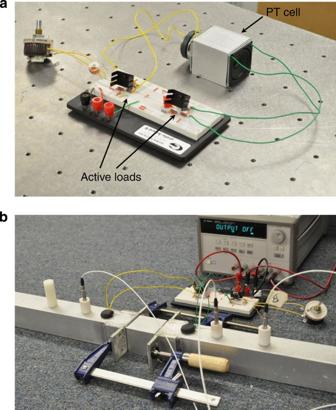Figure 4: Experiment. (a) Fabricated PT acoustic device showing the two loaded loudspeakers connected to distinct non-Foster electrical circuits. (b) The PT cell of panelais connected to two acoustic waveguides and the scattering parameters are measured. Figure 4: Experiment. ( a ) Fabricated PT acoustic device showing the two loaded loudspeakers connected to distinct non-Foster electrical circuits. ( b ) The PT cell of panel a is connected to two acoustic waveguides and the scattering parameters are measured. 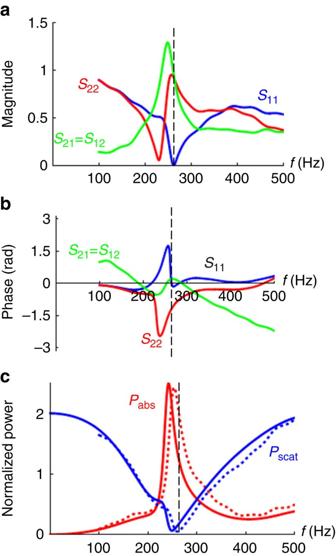Figure 5: Experimental results. (a,b) Measured scattering parameters, magnitude (a) and (b) phase. The device is unidirectionally transparent at the design frequency (dashed vertical line in all panels). (c) Absorbed power at the passive loudspeaker, and total scattered power by the device, normalized by the incident power at port 1, theory (solid lines) and experiment (dashed lines). Full size image Figure 5: Experimental results. ( a , b ) Measured scattering parameters, magnitude ( a ) and ( b ) phase. The device is unidirectionally transparent at the design frequency (dashed vertical line in all panels). ( c ) Absorbed power at the passive loudspeaker, and total scattered power by the device, normalized by the incident power at port 1, theory (solid lines) and experiment (dashed lines). Full size image Figure 5c shows the power absorbed (sensed) by the passive loudspeaker, obtained by measuring the sinusoidal voltage and current at the leads of the passive loudspeaker in the resistive circuit, and compared to the total power scattered by the device. Both quantities are normalized to the incident power. The experimentally measured curves (dashed) are in excellent agreement with analytical predictions (solid). Quite remarkably, the scattered power is extremely low around the design frequency, while the sensed power at the passive loudspeaker is twice the incident power, a direct proof of the negative power flow inside the device, consistent with our theoretical model. This proves the unique non-invasive nature of the fabricated sensing system, which can fully absorb the impinging signal, as well as its exact replica produced by the lasing portion of the sensor, while at the same time being invisible. Beyond proving the possibility of realizing an ideal invisible sensor, the results of Fig. 5 constitute experimental evidence of unidirectional transparency in a truly PT-symmetric metamaterial device, in contrast to previous experiments of unidirectionally reflecting structures with asymmetric loss distribution but without gain [23] . While this work has focused on a unidirectional sensing system in order to experimentally validate the ATR phenomenon, the same PT-symmetric topology can be readily used to form a bidirectional invisible sensor, if the acoustic distance is chosen to be a multiple of π ( Supplementary Note 4 ). Our results also demonstrate the general concept of pairing coherent lasing and coherent absorption to realize stable and efficient invisible sensors, exemplified here for acoustic waves, but also valid for electromagnetic waves and light. In this context, the proposed device may be somewhat related to time-reversed acoustics [33] , based on which time-reversed sources may be used as acoustic sinks [34] with interesting connections with the present design. We have also demonstrated how non-Foster loading of acoustic transducers can lead to acoustic gain, a simple strategy that, unlike previously established methods [35] , [36] , does not employ active control sensors or feedback loops. More generally, we have shown in this paper that acoustic waves provide a fertile ground to study and apply the anomalous scattering properties of PT-symmetric systems. We believe that our experiment can open new directions for loss compensation in metamaterials, as the observed phenomena are totally loss-immune and fully linear. In this context, we have experimentally demonstrated the exciting possibility to realize PT-based, fully loss-immune negative-index acoustic propagation, without relying on bulk metamaterials or non-linear effects. In our experimental setup, the wave is normally incident on a single PT cell, but we envision 2D or 3D arrays of such inclusions that may negatively refract or focus acoustic waves, in the spirit of ref. 30 . This may find promising applications in loss-compensated sound focusing, loss-immune phase compensation, non-invasive subwavelength acoustic imaging and sensing. Design of the electrical loads and stability considerations We chose the design frequency to be equal to the resonance frequency of the loudspeaker f r =250 Hz. This slightly simplifies the design by cancelling the reactive part of the mechanical impedance of the loudspeaker. The electrical loads are designed to provide a normalized acoustic impedance of ±2 at this frequency, while ensuring stability of the acoustic system. To ensure stability, the poles ω p of the acoustic admittance (see Supplementary Note 5 for a derivation of the acoustic admittance of a loudspeaker) are systematically placed so that their imaginary part is positive, within reasonable margins. We detail in the following the design procedure. Design of the +R element To fulfill the unidirectional invisibility condition, the passive + R element must have Z ac =2 at the design frequency. Plugging this value in the expression for the acoustic impedance of a loaded loudspeaker ( Supplementary Note 5 , Supplementary equation (28) ) and solving for Z L , one gets the value that the electrical load must take at this particular frequency: The above equation, evaluated for our particular loudspeaker whose properties are given in Supplementary Table 1 , suggests the use of a negative resistor − R 1 in series with a negative inductor − L 1 . By applying the Routh criterion [37] , [38] to the denominator of the acoustic admittance Y ac , it is straightforward to show that such an RL-loaded system is stable as long as R 1 < R e and L 1 < L e . For the value of R 1 required here, the first inequality holds; however, the required value for the inductance sets the system on the verge of instability. To avoid this issue, we choose instead L 1 =0.95 L e . Such an approximation on the imaginary part of the required electrical impedance (4) is very good, as the slope of the imaginary part at ω s , ∂ Z L /∂ ω = L e , is small, and the inductive part of the circuit may even be completely dropped without significantly altering the synthesized acoustic impedance. The final electrical design, with a typical negative impedance converter topology based on an operational amplifier, is shown in Supplementary Fig. 3 . The values of the electrical components in the electrical loads are summarized in Supplementary Table 2 . Note that the electrical circuit is active, although the synthesized acoustic impedance is passive. This is because the voice coil of the loudspeaker is intrinsically lossy, and the electrical circuit has to compensate for a part of these ohmic losses to fulfill the condition Z ac =2. By choosing another loudspeaker, it may happen that only a purely positive resistance would be sufficient, as evident in (4). Design of the −R element The starting point is to calculate the required electrical impedance at the design frequency to yield Z ac =−2. Using again Supplementary equation (28) in Supplementary Note 5 , we obtain for the real part and for the imaginary part The − R element cannot be synthesized any longer with a negative RL circuit, because the required value for the resistor exceeds R e and would lead to an unstable acoustic admittance. This means that the dispersion of the load has to be tailored to reach equations (5) and (6) at f s , and at the same time be stable. For instance, one can use the following dispersion for the electrical load: where s = jω , and A , B , α and Ω are positive coefficients. Without the minus sign, (7) represents a stable electrical impedance that can be realized using only passive components, by plugging in parallel three loads: a capacitive branch with capacitance C 1 =1/ A , a series RL branch with a resistance of R 2 = B /(Ω 2 + B 2 / A 2 −2 αB / A ) and an inductance L 2 = A /(Ω 2 + B 2 / A 2 −2 αB / A ), and a resistive branch with resistance R 2 = A 2 /(2 αA − B ). In equation (7), we add the minus sign because at f s the targeted impedance value has negative real and imaginary parts (see equations (5) and (6)). This will require the use of a negative impedance converter in front of the previously discussed parallel load, turning it into a non-Foster element, as sketched in Supplementary Fig. 4 . Now we look for the values of A and B such that the real and imaginary parts of Z L in (7) match the required values (5) and (6). We obtain and Finally, we need to determine the remaining parameters α and Ω so that the impedance is stable. To do so, we substitute equations (8) and (9) into equation (7), and calculate the acoustic admittance 1/ Z ac using Supplementary Equation (28) in Supplementary Note 5 . After a lengthy but straightforward calculation, we obtain a rational fraction in s , whose denominator is a polynomial of order 5. By applying Routh–Hurwitz criterion on the denominator [38] , we numerically determine a range of values for α and Ω that ensures stability of the acoustic system. In particular, the values α =800 rad s −1 and Ω=1,650 rad s −1 provide stability with good margins. The required values for the electrical components are summarized in Supplementary Table 2 . As a result, we obtain reasonable values for all elements, realizable with off-the-shelf components. We also plot in Supplementary Fig. 5 the frequency poles f i of the acoustic admittance Y ac in the complex plane. The green dots represent the poles of the + R (sensing) inclusion, and the orange dots represents the ones of the − R inclusion. As evident in the figure, the imaginary part of all the poles is positive, and stability of the acoustic admittance of each inclusion is guaranteed by design. Full-wave simulations The full-wave simulations throughout the paper were performed using the finite-element software COMSOL Multiphysics, by coupling the electrical circuits module (which is used to exactly model the electrical circuits) to the acoustic module (which solves for the acoustic scattering problem). The coupling basically implements the transduction mechanism, via the Laplace force that acts on the moving coil and the additional electromotive force in the voice coil due to the motion of the electrical wire in the static magnetic field. The pressure difference between the two sides of the loudspeaker membrane is taken as a voltage source in the electrical circuit module. The electrical circuits module feeds back the value of the current in the voice coil, which determines the membrane velocity imposed as an internal boundary condition in the acoustic module, and influences the scattering. The two modules are fully coupled and solved at the same time. The model is terminated by scattering boundary conditions that also include the incident field. The waveguide walls are approximated as hard wall boundaries. The scattering parameters were determined in frequency domain by using the well-established microphone transfer function method [39] , solving for a set of frequencies between 0 and 500 Hz, by increments of 0.5 Hz. The results, shown in Supplementary Fig. 6 , are in excellent agreement with both analytical predictions and measurements ( Figs 3 and 4 ). Experimental setup A tunable electrical circuit was built to allow for fine tuning of the electrical components, which were chosen to have small, but obviously finite, electrical tolerances. Two Visaton FRWS-5 8 Ohms (2′′) were loaded with the electrical circuits set on the values calculated above and inserted transversely, on both sides of a 5.5-cm-long piece of a square aluminium waveguide, with 5 cm external cross-section and a wall thickness of 6 mm. Two longer waveguides were connected to the structures on both sides, then sealed and clamped to the device to avoid any acoustic leakage. The device was powered using an Agilent triple output power supply E3631A, which provided the 18 V symmetric bias for the operational amplifiers OPA 548T used in the negative impedance converters. The dominant mode of the waveguide was excited several wavelengths upstream in the excitation waveguide, and the reflection coefficient was measured using the two microphones transfer function method [39] . The waveguide on the receiver side is terminated by an acoustic load, either a low-reflecting long piece of melamine foam or a highly reflective aluminium wall. We determine the scattering parameters by measuring the reflection coefficient from these two loads when the device is absent, then when it is present with port 1 facing the excitation, and finally when port 2 faces the excitation. This measurement procedure and the S-parameter retrieval method is described in the next section. Calibration and measurements We indicate with l 1 the load formed by the combination of the receiver waveguide and the melamine foam; similarly, we indicate with l 2 the load formed by terminating the receiver waveguide by a hard wall. Γ j is the reflection coefficient measured from load l j alone, that is, when the PT-device is absent. R i,j is the reflection coefficient measured when the PT-device is inserted, with port i facing the excitation, and the receiver waveguide loaded by the load l j . Performing a straightforward calculation based on the scattering signal flow graph method, one gets four equations relating the scattering parameters of the device to the measured reflection coefficients: Since the device is reciprocal, S 12 = S 21 , and we can solve for the S -parameters as The reflection coefficients Γ j and R i,j were measured using two PCB 130E21 ICP microphones, connected to the Data Physics SignalCalc Ace Quattro USB data acquisition system. While each inclusion is stable by design, we made sure to avoid to work around the instability condition of the entire experimental set-up, which occurs whenever 1−Γ j S ii =0. The source loudspeaker was driven with a chirp signal with frequencies from 100 to 500 Hz, and the frequency resolution was set to 0.25 Hz. The data, collected in time domain, were Fourier transformed using a fast Fourier transform algorithm. For each measurement, 15 chirps were sent and an arithmetic average of these 15 runs was taken. From these measurements, the scattering parameters were retrieved using equations (14)–(16), , . How to cite this article: Fleury, R. et al . An invisible acoustic sensor based on parity-time symmetry. Nat. Commun. 6:5905 doi: 10.1038/ncomms6905 (2015).